Sos-mediated cross-activation of wild-type Ras by oncogenic Ras is essential for tumorigenesis Mammalian cells contain three closely related ras genes, H-ras , K-ras and N-ras . Although in a given tumour type, oncogenic mutations are selectively observed in only one of the ras genes, the acquisition of the transformed phenotype has been shown to require the contribution of the normal products of the other ras genes. Here we demonstrate that oncogenic K-Ras promotes the activation of wild-type H- and N-Ras. This activation is mediated by oncogenic K-Ras-dependent allosteric stimulation of Sos and confers a growth advantage to oncogenic K-Ras harbouring cancer cells. These findings underscore the complementary functions of oncogenic and wild-type Ras in tumour cells and identify a potential new targeting strategy for Ras-driven tumours. As bona fide members of the GTPase family, the functional output of Ras proteins depends on their GTP-binding status that is dictated by the counteracting actions of guanine nucleotide exchange factors (GEFs) and GTPase-activating proteins (GAPs) [1] . In the absence of oncogenic mutations that compromise the response of Ras to the action of GAPs, the pool size of GTP-bound Ras molecules is thought to be largely controlled by the action of GEFs. The Ras-specific GEF Son of Sevenless (Sos) has a key role in regulating Ras activity by catalysing the exchange of GTP for GDP [2] . We have previously reported the presence of an allosteric site on Sos that interacts preferentially with Ras-GTP [3] . This interaction augments the catalytic activity of Sos by affecting conformational changes that release it from its autoinhibited state [4] . As oncogenic Ras proteins are constitutively bound to GTP, their interaction with the allosteric site on Sos would be favoured [4] , [5] . Accordingly, it is plausible that the occupation of the allosteric site on Sos by oncogenic Ras would lead to the enhancement of Sos-mediated activation of wild-type (WT) Ras. In the present study, we sought to test this prediction in the context of cancer cells harbouring oncogenic K-Ras. We demonstrate that through its ability to allosterically stimulate Sos, oncogenic K-Ras activates WT H- and N-Ras. Moreover, Sos-mediated cross-activation of WT Ras by oncogenic K-Ras contributes to cancer cell growth in vitro and in vivo . These results ascribe to Sos a heretofore unappreciated role in controlling the growth potential of cancer cells transformed by oncogenic K-Ras. Oncogenic K-Ras activates WT Ras through Sos To examine the capacity of oncogenic K-Ras to activate WT Ras, we employed initially an ectopic expression system that affords the selective detection of oncogenic and WT Ras proteins through differential epitope tagging. As shown in Fig. 1a , the expression of oncogenic K-Ras induced a robust activation of H- and N-Ras. This effect was observed under serum-deprived conditions ruling out the contribution of an oncogenic Ras-dependent autocrine mechanism in which secreted growth factors would promote the activation of WT Ras [6] , [7] , [8] , [9] . We next asked whether the effect of oncogenic K-Ras on the levels of GTP-bound H-Ras could be mediated by Sos. Mammalian cells contain two Sos genes, Sos1 and Sos2 , which code for closely related proteins [2] , [10] . As Sos1 has been defined as the primary GEF for Ras in terms of both abundance and activation [11] , [12] , we focused our analysis on Sos1 (hereafter referred to as Sos). As illustrated in Fig. 1c , the enhancement of H-Ras GTP levels induced by oncogenic K-Ras was abrogated when the expression of endogenous Sos was suppressed by short hairpin RNA (shRNA)-mediated silencing. This effect was rescued by the expression of an shRNA-resistant Sos construct (*Sos WT ; Fig. 1c ), thus excluding the contribution of off-target silencing mechanisms and implicating Sos as an essential intermediate in the cross talk between oncogenic K-Ras and WT H-Ras. 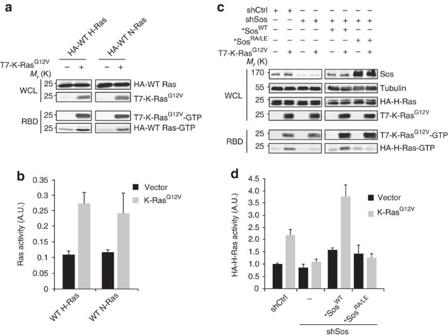Figure 1: Expression of oncogenic K-Ras promotes the activation of WT H-Ras through the allosteric stimulation of Sos. (a) HeLa cells were transfected with HA-tagged WT Ras isoforms either alone or with T7-tagged K-RasG12Vconstruct as indicated. Following serum starvation, the levels of GTP-bound WT and oncogenic Ras were determined by the RBD pull-down assay and were detected using anti-HA or anti-T7 antibodies, respectively. (b) The levels of activated Ras were quantified by densitometry scanning and normalized to the total levels of the respective isoform. Values are means±s.d. from three independent experiments. (c) HeLa cells were transfected with pSUPER constructs expressing scrambled shRNA (shCtrl) or shRNA targeting Sos (shSos). Cells were selected with blasticidin S for 3 days and then transfected with HA-H-Ras and, as indicated, T7-K-RasG12Vconstructs in the absence or presence of shRNA-resistant WT or RA/LE Sos constructs (*SosWTand *SosRA/LE). Following serum starvation for 20 h, the levels of GTP-bound HA-H-Ras and T7-K-Ras were determined by the RBD pull-down assay and were detected using anti-HA and anti-T7 antibodies, respectively. (d) Quantification of H-Ras-GTP was carried out by densitometry scanning and data was normalized to the levels of total HA-H-Ras. Values are means±s.d. from three independent experiments presented as fold activation compared with shCtrl vector. For all panels, the efficiency of Sos suppression was analysed by western blotting and tubulin was used as a loading control. WCL, whole cell lysate; A.U., arbitrary units. Figure 1: Expression of oncogenic K-Ras promotes the activation of WT H-Ras through the allosteric stimulation of Sos. ( a ) HeLa cells were transfected with HA-tagged WT Ras isoforms either alone or with T7-tagged K-Ras G12V construct as indicated. Following serum starvation, the levels of GTP-bound WT and oncogenic Ras were determined by the RBD pull-down assay and were detected using anti-HA or anti-T7 antibodies, respectively. ( b ) The levels of activated Ras were quantified by densitometry scanning and normalized to the total levels of the respective isoform. Values are means±s.d. from three independent experiments. ( c ) HeLa cells were transfected with pSUPER constructs expressing scrambled shRNA (shCtrl) or shRNA targeting Sos (shSos). Cells were selected with blasticidin S for 3 days and then transfected with HA-H-Ras and, as indicated, T7-K-Ras G12V constructs in the absence or presence of shRNA-resistant WT or RA/LE Sos constructs (*Sos WT and *Sos RA/LE ). Following serum starvation for 20 h, the levels of GTP-bound HA-H-Ras and T7-K-Ras were determined by the RBD pull-down assay and were detected using anti-HA and anti-T7 antibodies, respectively. ( d ) Quantification of H-Ras-GTP was carried out by densitometry scanning and data was normalized to the levels of total HA-H-Ras. Values are means±s.d. from three independent experiments presented as fold activation compared with shCtrl vector. For all panels, the efficiency of Sos suppression was analysed by western blotting and tubulin was used as a loading control. WCL, whole cell lysate; A.U., arbitrary units. Full size image Allosteric stimulation of Sos by oncogenic K-Ras Under normal growth conditions, the activation of Ras proteins by Sos is an inducible process that is triggered by receptor–ligand interactions [13] , [14] , [15] , [16] . However, the dependence of H-Ras activation by oncogenic K-Ras on Sos was observed under serum-deprivation conditions suggesting that the Sos-mediated cross-activation of WT Ras by oncogenic Ras takes place at the post-receptor level and could involve the engagement of the allosteric site of Sos by oncogenic K-Ras. To test this idea, we took advantage of a Sos mutant shown previously to be defective in Ras-GTP binding at the allosteric site (*Sos RA/LE ) [4] . In contrast to *Sos WT , the introduction of *Sos RA/LE into cells in which endogenous Sos expression was silenced failed to reconstitute oncogenic K-Ras-induced activation of WT H-Ras ( Fig. 1c ). These results support the postulation that oncogenic Ras can upregulate the level of activity of WT Ras by allosteric stimulation of Sos. To determine whether the interaction of constitutively active K-Ras with the Sos allosteric site is required for WT H-Ras activity in the setting of tumour cells harbouring an oncogenic K-Ras allele, we carried out the Sos knockdown/rescue experiments in pancreatic cancer cell lines. As demonstrated in Fig. 2a , in serum-deprived MIA PaCa-2 cells, the suppression of Sos expression was associated with a pronounced decrease in H-Ras-GTP levels. The reconstitution of *Sos WT into the knockdown cells was sufficient to restore H-Ras activity whereas the expression of *Sos RA/LE was without an effect on H-Ras-GTP levels. Significantly, the capacity of *Sos WT to reinstate H-Ras-GTP levels was abolished when oncogenic K-Ras expression was suppressed, underscoring the dependence of Sos on oncogenic Ras for the activation of WT Ras in cancer cells ( Fig. 2c ). Together, these results identify Sos as a molecular scaffold for WT and oncogenic Ras proteins, and indicate that this scaffold function is utilized by oncogenic Ras to modulate the activity of WT Ras. 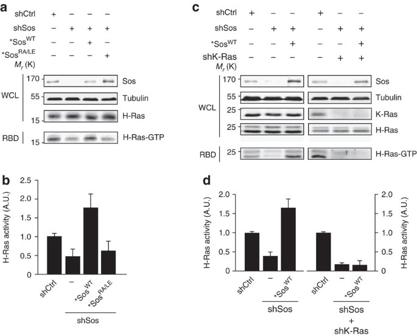Figure 2: Oncogenic K-Ras-dependent activation of WT H-Ras is mediated by the allosteric stimulation of Sos. (a) MIA PaCa-2 cells stably expressing inducible miR-30-based shCtrl or shSos were infected with lentiviral inducible *SosWTor *SosRA/LE. Following doxycycline treatment, cells were serum-starved for 20 h and H-Ras-GTP levels were measured using the RBD pull-down assay. (b) The levels of activated Ras were quantified by densitometry scanning and normalized to the levels of total H-Ras. Values are means±s.d. from three independent experiments presented as fold activation compared with shCtrl. (c) MIA PaCa-2 cells stably expressing inducible miR-30-based shCtrl or shSos were infected with lentiviral inducible *SosWTin the presence or absence of shK-Ras. H-Ras-GTP levels were measured using the RBD pull-down assay. (d) The levels of activated Ras were quantified by densitometry scanning and normalized to the levels of total H-Ras. Values are means±s.d. from three independent experiments presented as fold activation compared with shCtrl. For all panels, the efficiency of Sos suppression was analysed by western blotting and tubulin was used as a loading control. WCL, whole cell lysate; A.U., arbitrary units. Figure 2: Oncogenic K-Ras-dependent activation of WT H-Ras is mediated by the allosteric stimulation of Sos. ( a ) MIA PaCa-2 cells stably expressing inducible miR-30-based shCtrl or shSos were infected with lentiviral inducible *Sos WT or *Sos RA/LE . Following doxycycline treatment, cells were serum-starved for 20 h and H-Ras-GTP levels were measured using the RBD pull-down assay. ( b ) The levels of activated Ras were quantified by densitometry scanning and normalized to the levels of total H-Ras. Values are means±s.d. from three independent experiments presented as fold activation compared with shCtrl. ( c ) MIA PaCa-2 cells stably expressing inducible miR-30-based shCtrl or shSos were infected with lentiviral inducible *Sos WT in the presence or absence of shK-Ras. H-Ras-GTP levels were measured using the RBD pull-down assay. ( d ) The levels of activated Ras were quantified by densitometry scanning and normalized to the levels of total H-Ras. Values are means±s.d. from three independent experiments presented as fold activation compared with shCtrl. For all panels, the efficiency of Sos suppression was analysed by western blotting and tubulin was used as a loading control. WCL, whole cell lysate; A.U., arbitrary units. Full size image An anticipated corollary of the mechanism described above is that the activity status of WT Ras isoforms would be dependent upon the presence of a mutant isoform. Accordingly, we have found that the silencing of K-Ras expression in pancreatic (AsPC-1, Fig. 3a ; MIA PaCa-2, Fig. 3c ; and PL45, Fig. 3e–h ) and colon (HCT-116, Fig. 3i ) cancer cells harbouring an oncogenic mutation in this allele was accompanied by a reduction in the levels of GTP-bound H-Ras ( Fig. 3a–f ). N-Ras GTP levels were subject to the same downregulation following the silencing of K-Ras expression ( Fig. 3g ). Although the silencing construct that we have used does not discriminate between the WT and oncogenic alleles of K-Ras, the fact that the suppression of K-Ras expression produced the same effect in cells in which the WT allele of K-Ras is deleted (MIA PaCa-2) is consistent with the loss of function of oncogenic K-Ras being the principle contributor to the observed biochemical phenotype. That the attenuation of H-Ras activity does not reflect an overall reduction in signalling capabilities owing to the loss of oncogene expression is indicated by our observation from two independent cell lines that ligand-mediated activation of epidermal growth factor receptor (EGFR) and its downstream effector PLCγ are unaffected by the suppression of oncogenic K-Ras expression ( Fig. 3k ; Supplementary Fig. S1 ). Consistent with the postulated role of Sos allosteric modulation by oncogenic K-Ras in dictating the activity of WT H-Ras, the interdependence between oncogenic K-Ras and WT H-Ras was observed in the absence of serum growth factors as all experiments were carried out in cells maintained in serum-free medium. The lack of significant contribution of receptor-mediated activation of WT HRas to its overall GTP-binding levels is also indicated by the fact that growth factor deprivation had no effect on H-Ras activity ( Fig. 3m ). Together, these observations implicate oncogenic K-Ras in regulating the activity of WT Ras proteins in cancer cells. 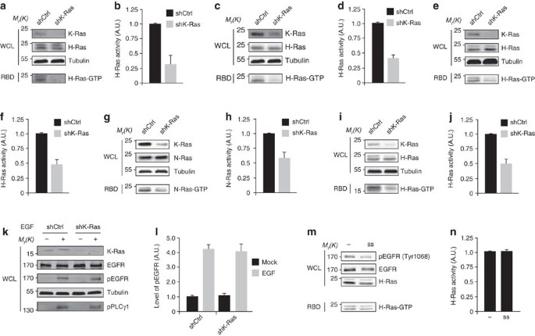Figure 3: The activity of WT H-Ras is dependent on oncogenic K-Ras. (a–j) Cancer cell lines harbouring oncogenic K-Ras derived from pancreas (AsPC-1 (a,b), MIA PaCa-2 (c,d) and PL45 (e–h)) or colon (HCT-116 (i,j)) were infected with lentiviral tetracycline-inducible miR30-based scrambled shRNA (shCtrl) or K-Ras shRNA (shK-Ras). Following doxycycline treatment, cells were serum-starved for 20 h, and the levels of GTP-bound H-Ras (a-f,i,j) or N-Ras (g,h) were determined by the RBD pull-down assay as described in Methods. The efficiency and specificity of knockdown were analysed by immunoblotting with anti-K-, H- or N-Ras antibodies. Quantification of the levels of activated H-Ras (b,d,f,j) or activated N-Ras (h) was done by densitometry scanning and normalized to the levels of total H-Ras or N-Ras, respectively. Values are means±s.d. from three independent experiments presented as fold activation compared with shCtrl. (k) MIA PaCa-2 cells engineered to express shCtrl or shK-Ras as described in (a–j) were serum-starved for 20 h and then stimulated with 50 ng ml−1EGF for 10 min at 37 °C. Activation of EGFR signalling was determined by western blotting using anti-phospho-EGFR (Tyr1068) and anti-phospho-PLCγ1 (Tyr783) antibodies. (l) Quantification of the levels of activated EGFR in (k) was done by densitometry scanning and normalized to the levels of total EGFR. Values are means±s.d. from three independent experiments presented as fold activation compared with shCtrl (mock). (m) MIA PaCa-2 cells were either cultured in full-serum media (−) or starved by frequent replenishment of serum-free media (ss; changed every 2 h for a total 16 h). Cell lysates were probed with the specified antibodies. (n) The levels of GTP-bound H-Ras in (m) were determined by RBD pull-down and quantified by densitometry scanning and normalized to the total levels of H-Ras. Values are means±s.d. from three independent experiments presented as fold activation compared with full serum media (−). For all panels, tubulin was used as loading control. WCL, whole cell lysate; A.U., arbitrary units. Figure 3: The activity of WT H-Ras is dependent on oncogenic K-Ras. ( a – j ) Cancer cell lines harbouring oncogenic K-Ras derived from pancreas (AsPC-1 ( a,b ), MIA PaCa-2 ( c,d ) and PL45 ( e – h )) or colon (HCT-116 ( i,j )) were infected with lentiviral tetracycline-inducible miR30-based scrambled shRNA (shCtrl) or K-Ras shRNA (shK-Ras). Following doxycycline treatment, cells were serum-starved for 20 h, and the levels of GTP-bound H-Ras ( a-f,i,j ) or N-Ras ( g,h ) were determined by the RBD pull-down assay as described in Methods. The efficiency and specificity of knockdown were analysed by immunoblotting with anti-K-, H- or N-Ras antibodies. Quantification of the levels of activated H-Ras ( b,d,f,j ) or activated N-Ras ( h ) was done by densitometry scanning and normalized to the levels of total H-Ras or N-Ras, respectively. Values are means±s.d. from three independent experiments presented as fold activation compared with shCtrl. ( k ) MIA PaCa-2 cells engineered to express shCtrl or shK-Ras as described in ( a – j ) were serum-starved for 20 h and then stimulated with 50 ng ml −1 EGF for 10 min at 37 °C. Activation of EGFR signalling was determined by western blotting using anti-phospho-EGFR (Tyr1068) and anti-phospho-PLCγ1 (Tyr783) antibodies. ( l ) Quantification of the levels of activated EGFR in ( k ) was done by densitometry scanning and normalized to the levels of total EGFR. Values are means±s.d. from three independent experiments presented as fold activation compared with shCtrl (mock). ( m ) MIA PaCa-2 cells were either cultured in full-serum media (−) or starved by frequent replenishment of serum-free media (ss; changed every 2 h for a total 16 h). Cell lysates were probed with the specified antibodies. ( n ) The levels of GTP-bound H-Ras in ( m ) were determined by RBD pull-down and quantified by densitometry scanning and normalized to the total levels of H-Ras. Values are means±s.d. from three independent experiments presented as fold activation compared with full serum media (−). For all panels, tubulin was used as loading control. WCL, whole cell lysate; A.U., arbitrary units. Full size image Sos contributes to cancer cell growth and signalling Given the reported contribution of WT Ras isoforms to the transformed phenotype of cancer cells harbouring oncogenic Ras [17] , [18] , we set out to investigate the significance of Sos-dependent activation of WT Ras by oncogenic Ras for cancer cell growth. To this end, we first monitored the effect of Sos silencing on the growth characteristics of oncogenic K-Ras-harbouring cells in culture. The loss of Sos function in MIA PaCa-2 cells maintained in serum-deprived growth medium was associated with a marked decrease in cell expansion ( Fig. 4a–d ). A similar effect was observed in PL45, CFPAC-1 and AsPC-1 cell lines ( Supplementary Fig. S2 ), suggesting that the dependency on Sos for cancer cell growth might represent a general feature of cancer cells harbouring oncogenic Ras. In support of this idea, BxPC-3 and Hs700T cell lines, which harbour only WT Ras proteins, were essentially resistant to the deleterious effect of Sos knockdown on cell growth ( Supplementary Fig. S3 ). 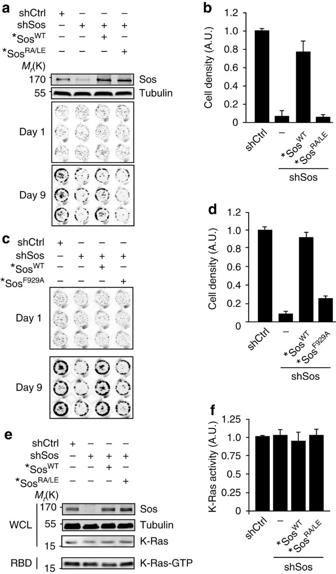Figure 4: Sos-mediated cross-activation of WT Ras by oncogenic K-Ras contributes to pancreatic cancer cell growth. (a–d) MIA PaCa-2 cells engineered as inFig. 2ato express inducible shCtrl, shSos, *SosWTand *SosRA/LE(a,b) or *SosF929A(c,d) as indicated were cultured in 0.5% serum in the presence of doxycycline for the time indicated. Efficiency of knockdown and ectopic expression of Sos were confirmed by western blotting. Tubulin was used as a loading control. Cell densities were determined by Syto60 staining and quantified (b,d) as described in Methods. Values are means±s.d. of technical triplicates presented as fold activation compared with shCtrl. The experiment shown is representative of three independent experiments. (e,f) Oncogenic K-Ras activity does not depend on the expression of Sos. (e) The levels of K-Ras-GTP in serum-deprived MIA PaCa-2 cells harbouring the indicated constructs were determined by the RBD pull-down assay. Tubulin was used as a loading control. WCL, whole cell lysate. (f) The levels of activated Ras were quantified by densitometry scanning and normalized to the total levels of K-Ras. Values are means±s.d. from three independent experiments presented as fold activation compared with shCtrl. A.U., arbitrary units. Figure 4: Sos-mediated cross-activation of WT Ras by oncogenic K-Ras contributes to pancreatic cancer cell growth. ( a – d ) MIA PaCa-2 cells engineered as in Fig. 2a to express inducible shCtrl, shSos, *Sos WT and *Sos RA/LE ( a,b ) or *Sos F929A ( c,d ) as indicated were cultured in 0.5% serum in the presence of doxycycline for the time indicated. Efficiency of knockdown and ectopic expression of Sos were confirmed by western blotting. Tubulin was used as a loading control. Cell densities were determined by Syto60 staining and quantified ( b,d ) as described in Methods. Values are means±s.d. of technical triplicates presented as fold activation compared with shCtrl. The experiment shown is representative of three independent experiments. ( e,f ) Oncogenic K-Ras activity does not depend on the expression of Sos. ( e ) The levels of K-Ras-GTP in serum-deprived MIA PaCa-2 cells harbouring the indicated constructs were determined by the RBD pull-down assay. Tubulin was used as a loading control. WCL, whole cell lysate. ( f ) The levels of activated Ras were quantified by densitometry scanning and normalized to the total levels of K-Ras. Values are means±s.d. from three independent experiments presented as fold activation compared with shCtrl. A.U., arbitrary units. Full size image Oncogenic Ras proteins are stabilized in the GTP-bound form owing to their insensitivity to the action of GAPs [19] . Consistent with this mode of regulation, the levels of GTP-bound oncogenic K-Ras in MIA PaCa-2 cells were not affected by the suppression of Sos expression ( Fig 4e ), indicating that the compromised cell growth observed under these conditions cannot be attributed to a reduction in K-Ras-dependent oncogenic output. Furthermore, the growth defect displayed by Sos-deficient MIA PaCa-2, CFPAC-1, AsPC-1 or PL45 cells could be rescued by the re-expression of *Sos WT but not *Sos RA/LE ( Fig. 4a ; Supplementary Fig. S2 ). The expression of neither *Sos WT nor *Sos RA/LE altered the levels of GTP-bound oncogenic Ras ( Fig. 4e ). In light of our finding that the allosteric stimulation of Sos by oncogenic Ras upregulates the activity of WT Ras ( Fig. 2a–d ), the differential rescuing capacity of *Sos WT and *Sos RA/LE indicates that the requirement for Sos to support cancer cell growth relates to its role in mediating the activation of WT Ras by oncogenic Ras. In support of this interpretation, the rescuing capacity of *Sos WT was abrogated by the introduction of a mutation shown to impair the catalytic activity of Sos (F929A, ref. 20 ) ( Fig. 4c ). The two major Ras effector pathways that control cell proliferation and survival are Raf-MEK-ERK and PI3-K-AKT, respectively [21] , [22] . The suppression of Sos expression in MIA PaCa-2 and PL45 cells was associated with reduced signalling through the ERK-MAPK signalling axis as indicated by the decrease in the levels of phosphorylated MAP-kinase kinase (MEK) and extracellular signal-regulated kinase (ERK) ( Fig. 5a–d ; Supplementary Fig. S4a,b ). The compromised ERK-MAPK signalling capacity in these cells was further indicated by a pronounced reduction in the levels of phosphorylated S6 ( Fig. 5a ; Supplementary Fig. S4a ), the substrate of S6 kinase, which is an ERK-mTORC1 target [23] . In contrast, the activity of the PI3-K-AKT axis was unaffected by the status of Sos expression. Indeed, the sensitivity of ERK-MAPK signalling to the loss of Sos function is consistent with the observed growth impediment of pancreatic cancer cells lacking Sos ( Fig. 5e and Supplementary Fig. S4c ). The impaired ERK-MAPK signalling axis in Sos-deficient cells was rescued by expression of *Sos WT but not *Sos RA/LE ( Fig. 5a ; Supplementary Fig. S4a ) confirming that the alteration of signalling resulting from Sos suppression reflects the impaired activation through the allosteric stimulation of WT Ras by Sos. Significantly, the inhibitory effect of Sos depletion on signalling was completely rescued by the expression of H-Ras G12V affirming the link between the GTP-binding status of H-Ras and the ERK-S6 signalling profile in cells harbouring oncogenic K-Ras ( Fig. 5c ). Similarly, N-Ras G12D rescued the inhibitory effect of Sos depletion on signalling indicating that this is not an isoform-specific effect ( Supplementary Fig. S5 ). Together, the observation that ERK signalling in cells expressing oncogenic Ras can be manipulated by altering Sos levels represents a departure from the widely held notion that the output of this signalling axis is predominantly dictated by the activity of the oncogenic allele of Ras. Rather, our findings lend support to the idea that the Ras signalling landscape in cancer cells transformed by oncogenic Ras reflects the mutual contribution of the WT and oncogenic alleles. 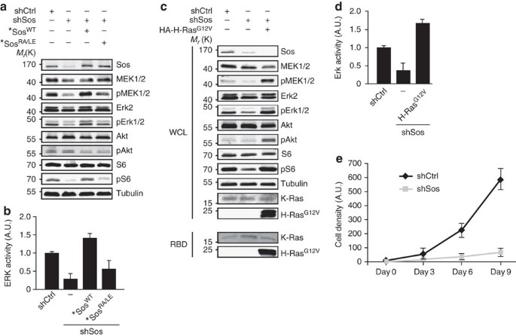Figure 5: Sos-mediated cross-activation of WT Ras by oncogenic K-Ras contributes to pancreatic cancer cell signalling. (a–d) MIA PaCa-2 cells that were engineered as inFig. 2ato express inducible shCtrl, shSos and *SosWTor *SosRA/LE(a,b) or HA-H-RasG12V(c,d) were cultured in 0.5% serum in the presence of doxycycline. Cells were lysed, immunoblotted and probed with the specified antibodies. WCL, whole cell lysate. Values (b,d) of ERK activity are presented as fold activation compared with shCtrl and represent means±s.d. from three independent experiments. A.U., arbitrary units. (e) Effect of suppression of Sos expression on the kinetics of pancreatic cancer cell growth. MIA PaCa-2 cells expressing shCtrl or shSos were maintained in culture for the indicated intervals. Cell density at each time point was analysed by Syto60 staining. Values are means±s.d. from three independent experiments. A.U., arbitrary units. Figure 5: Sos-mediated cross-activation of WT Ras by oncogenic K-Ras contributes to pancreatic cancer cell signalling. ( a – d ) MIA PaCa-2 cells that were engineered as in Fig. 2a to express inducible shCtrl, shSos and *Sos WT or *Sos RA/LE ( a,b ) or HA-H-Ras G12V ( c,d ) were cultured in 0.5% serum in the presence of doxycycline. Cells were lysed, immunoblotted and probed with the specified antibodies. WCL, whole cell lysate. Values ( b,d ) of ERK activity are presented as fold activation compared with shCtrl and represent means±s.d. from three independent experiments. A.U., arbitrary units. ( e ) Effect of suppression of Sos expression on the kinetics of pancreatic cancer cell growth. MIA PaCa-2 cells expressing shCtrl or shSos were maintained in culture for the indicated intervals. Cell density at each time point was analysed by Syto60 staining. Values are means±s.d. from three independent experiments. A.U., arbitrary units. Full size image Sos is required for tumour growth An intriguing possibility raised by the deleterious effect of Sos suppression on pancreatic cancer cell growth is that Sos function is required to support tumorigenic growth. To test this prediction, MIA PaCa-2 cell lines expressing control silencing vector or Sos silencing vector alone or with *Sos WT , *Sos RA/LE or *Sos F929A were injected into nude mice and tumour growth was monitored over time. As demonstrated in Fig. 6a and Supplementary Fig. S6 , tumour formation was nearly abolished in cells depleted of Sos and this effect could be rescued by complementation with *Sos WT but not *Sos RA/LE or *Sos F929A . Consistent with the signalling profile observed in the cell growth experiments, the silencing of Sos expression had no effect on K-Ras GTP levels but was accompanied by a significant reduction in ERK activity ( Fig. 6c ). Furthermore, the suppressive effect of Sos silencing on the in vivo growth of MIA PaCa-2 cells was associated with a marked decrease in cell proliferation ( Fig. 6e ). Together, these observations indicate that Sos-dependent activation of WT Ras by oncogenic Ras is required for tumorigenesis. 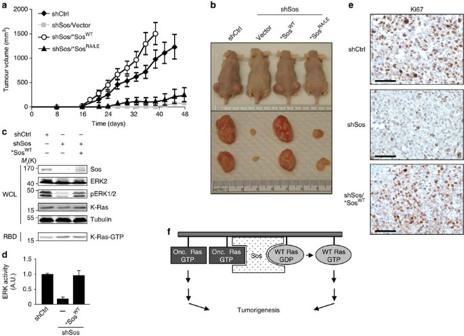Figure 6: Sos-mediated cross-activation of WT Ras by oncogenic K-Ras is required for tumour growth. (a) MIA PaCa-2 cells harbouring the indicated inducible constructs were injected subcutenously into mice. Following injections, animals were fed doxycycline-containing diet and tumour growth was measured as described in Methods. Values are means±s.d. from three independent experiments. (b) Representative mice and tumours are shown. (c) Signalling analysis of the indicated xenografts. ERK activity was assessed by immunoblotting for pERK and K-Ras-GTP levels were determined by RBD pull down. Tubulin was used as a loading control. (d) Values of ERK activity are presented as fold activation compared with shCtrl and represent means±s.d. from three independent experiments. (e) Cell proliferation of the indicated xenografts as assessed by immunohistochemical staining for Ki-67. Images shown are representative of three independent experiments. Scale bars, 50 μm. (f) Schematic depiction of the role of Sos in oncogenic Ras-driven tumorigenesis. The binding of oncogenic Ras (Onc.) to the allosteric site promotes the activation of WT Ras. The signalling output of both forms of Ras is required for tumorigenesis. Figure 6: Sos-mediated cross-activation of WT Ras by oncogenic K-Ras is required for tumour growth. ( a ) MIA PaCa-2 cells harbouring the indicated inducible constructs were injected subcutenously into mice. Following injections, animals were fed doxycycline-containing diet and tumour growth was measured as described in Methods. Values are means±s.d. from three independent experiments. ( b ) Representative mice and tumours are shown. ( c ) Signalling analysis of the indicated xenografts. ERK activity was assessed by immunoblotting for pERK and K-Ras-GTP levels were determined by RBD pull down. Tubulin was used as a loading control. ( d ) Values of ERK activity are presented as fold activation compared with shCtrl and represent means±s.d. from three independent experiments. ( e ) Cell proliferation of the indicated xenografts as assessed by immunohistochemical staining for Ki-67. Images shown are representative of three independent experiments. Scale bars, 50 μm. ( f ) Schematic depiction of the role of Sos in oncogenic Ras-driven tumorigenesis. The binding of oncogenic Ras (Onc.) to the allosteric site promotes the activation of WT Ras. The signalling output of both forms of Ras is required for tumorigenesis. Full size image The collaboration between oncogenic and WT Ras proteins in promoting the transformed phenotype has been documented in multiple settings and has been attributed predominantly to the distinct but complementary signalling activities of different Ras isoforms [17] , [18] , [24] , [25] , [26] . By its very nature this heterotypic collaboration is distinct from the antagonistic effects on oncogenic K-Ras and N-Ras ascribed to WT K-Ras [27] , [28] and NRas [29] , respectively. The present study identifies a previously undescribed mechanism for the co-option of WT Ras proteins by the oncogenic protein which, on the basis of previous structural and biochemical studies [3] , [30] , most likely involves the tri-molecular interaction between oncogenic Ras, Sos and WT Ras ( Fig. 6f ). Each interface of this interaction, namely the allosteric site and the catalytic site of Sos, can in principle be equally recognized by all Ras isoforms with the only provision being that oncogenic Ras would be the preferred ligand for the allosteric site. Thus, this mechanism would be broadly applicable to tumour cells harbouring different oncogenic alleles of Ras and should permit the combinatorial activation of all Ras isoforms. Furthermore, the essential role that this Sos-mediated cross-activation mechanism plays in tumorigenesis points to a cancer cell vulnerability that might be amenable to therapeutic targeting. General reagents Epidermal growth factor (EGF) was from Invitrogen. Glutathione Sepharose was from GE Healthcare. The antibodies used for immunohistochemistry and western blot analyses were from the following sources: anti-HA 12CA5 and anti-Sos1 (C-terminus) were from Upstate; anti-T7 was from Novagen; anti-EGFR, anti-H-Ras (C-20), anti-N-Ras (F155) and anti-K-Ras (F234) were from Santa Cruz; anti-tubulin was from Sigma; anti-MEK1/2, anti-phospho-MEK1/2 (Ser217/221), anti-ERK2, anti-phospho-ERK1/2 (Thr202/Tyr204), anti-AKT, anti-phospho-AKT (Ser473), anti-S6, anti-phospho-S6 (Ser240/244) and anti-phospho-EGFR (Tyr1068) were purchased from Cell Signaling; anti-Ki-67 was from Vector Labs; and phospho-PLCγ1 (Tyr783) was a kind gift from Dr Mark Philips. Plasmids Mammalian expression vectors of pCGT-K-Ras G12V , pCGN-H-Ras G12V , pCGT-N-Ras G12D and pCGN-H-Ras and N-Ras isoforms have been previously described [30] . The constructs for RNA interference were generated with either the pcDNA6/SUPER vector (a kind gift from Dr Gwuanwei Du, University of Texas at Houston) [30] or constructed into the doxycycline-inducible version of pTRIPZ according to the manufacturer’s protocol (Open Biosystems). The oligonucleotides used for cloning contained the following target sequences or scrambled sequence (shCtrl): for shSos (targets both hSos1 and hSos2), 5′-GACAGTGTTGTAATGAATT-3′; for shK-Ras, 5′-GGAGGGCTTTCTTTGTGTATTT-3′; and for shCtrl, 5′-GGCAGATACTCTGATAAAT-3′. The shRNA-resistant full-length Sos constructs were generated by introducing the following nucleotide substitutions (underlined) into the Sos sequence and cloned into pCGN vector or the doxycycline-inducible pLenti CMV/TO vector (Addgene): for *Sos RA/LE , 5′-CAGCCTGTGCAA GA G GC AGTATTAAATGTATGTCGG-3′; for *Sos WT , 5′- GAAAAGACATTGG G CA A TG C TG C AA C GA G TTTATAATGGAAGG-3′; and for *Sos F929A , 5′-CCACCATGTGTGCCT GCC TTTGGAATTTATCTC-3′. Cell culture transfection and lentiviral infection HeLa cells, human pancreatic cancer cell lines MIA PaCa-2 (KRas 34G>T), BxPC-3 (KRas, no mutation), Hs700T (KRas, no mutation), PL45 (KRas 35G>A), CFPAC-1 (KRas 35G>T) and AsPC-1 (KRas 35G>A), and the colon cancer cell line HCT-116 (KRas 38G>A) were cultured as specified by ATCC (Manassas, VA, USA). For transient expression in HeLa cells, transfection of pSUPER constructs of scrambled (shCtrl) or shSos were performed with Lipofectamine 2000 (Invitrogen) according to the manufacturer’s directions. After 24 h of expression, the media was replaced with fresh media supplemented with 10 μg ml −1 Blasticidin (Invitrogen). Three days after selection, cells were cotransfected with Ras or Sos as indicated. After 16 h of expression, the cells were serum-starved for 20 h and then collected. Generation of lentivirus was done according to standard protocols. Briefly, 293T cells were plated in a 10-cm dish for 12–16 h. One hour before transfection by the calcium phosphate method, media was replaced with fresh media. Twenty micrograms of lentiviral vector, 13 μg of packaging vector and 7 μg of envelope plasmid were diluted into 500 μl 2XHBS (0.28M sodium chloride, 0.05 M HEPES (4-(2-hydroxyethyl)-1-piperazineethanesulfonic acid), 1.5 mM Na 2 HPO 4 , pH 7.0). While gently vortexing this solution, 500 μl of 0.25 M calcium chloride was added, dropwise, over a period of 1 min. The mixture was incubated for 20 min. All solutions and steps were at room temperature. The DNA precipitate was then added slowly, dropwise, to the cells and incubated at 37 °C, 5% CO 2 , for 7 h at which time the complex was aspirated and 9 ml of fresh media was added. The next day the virus-containing media was collected and stored at 4 °C. Six millilitres of fresh media was added. The next day, the virus-containing media was collected, pooled with that of the previous day, centrifuged at 2,500 r.p.m., filtered through a 0.45 μm syringe and concentrated using a 100-kDa molecular weight cutoff Amicon filter (Millipore). Aliquots were stored at −80 °C. For knockdown experiments in MIA PaCa-2, BxPC-3, PL45, AsPC-1 and HCT-116 cells, cells were infected (multiplicity of infections for cell lines: Mia PaCa-2, 5; all others, 10) with pTripz constructs of shCtrl, shSos or shK-Ras and selected with puromycin (Calbiochem; for AsPC-1, 4 μg ml −1 ; for all others, 2 μg ml −1 ) for 4 days. Where indicated in the figures, lentiviral *Sos WT , *Sos RA/LE or *Sos F929A or HRas G12V constructs were then transduced. shRNA and Sos expression were induced for 3 days with doxycycline (2 μg ml −1 ; Sigma). The cells were serum-starved for 20 h before analysis. Ras activity assay and immunoblot analysis The levels of active, GTP-loaded Ras were determined by GST-Raf-RBD pull-down assay. In brief, GST–Raf–RBD fusion proteins expressed in Escherichia coli were purified by incubation with glutathione agarose beads. Cells were collected in RBD lysis buffer containing 25 mM Tris-HCl (pH 7.4), 120 mM NaCl, 10 mM MgCl 2 , 1 mM EDTA, 10% glycerol, 10 μg ml −1 pepstatin, 50 mM NaF, 1% aprotinin, 10 μg ml −1 leupeptin, 1 mM Na 3 VO 4 , 10 mM benzamidine, 10 μg ml −1 soybean trypsin inhibitor, 1% NP40 and 0.25% sodium deoxycholic acid. The samples were then centrifuged, and supernatants were incubated with 20 μg GST-Raf-RBD immobilized beads for 1.5 h at 4 °C. Bound proteins were eluted with SDS sample buffer, separated by SDS-15% polyacrylamide gel electrophoresis and transferred to nitrocellulose membrane. The proteins were detected by immunoblotting with the indicated antibodies. The levels of Ras activation, phospho-MEK1/2, phospho-ERK, phospho-S6, phospho-AKT, phospho-EGFR, phospho-PLCγ1, Sos1 or tubulin were determined using the Odyssey infrared system (Li-Cor). Relative ERK phosphorylation or Ras activation was quantified by Odyssey V2.1 software (Li-Cor) and normalized to ERK or Ras expression. Cell growth assay The cell growth assay was carried out by nucleic acid staining with Syto60 (Invitrogen) dye. Cells were prepared to express inducible shRNA and Sos as described above. Cells were treated with doxycycline for 3 days then equal cell numbers were plated in 96-well plates and maintained in doxycycline. At the times indicated, cells were fixed with 3.7% formaldehyde for 20 min, washed three times with PBS, permeabilized with 0.1% triton X-100 (in PBS) for 5 min and blocked with 0.1% bovine serum albumin (in PBS) for 5 min. Cells were then stained with 1 μM Syto60 dye (prepared in block solution) for 1 h in the dark. Cells were washed twice with PBS. All steps were carried out at room temperature. Fluorescence was quantified using the Odyssey infrared system (Li-Cor) in the IR700 channel. Cells were harvested for western blot analysis. Athymic nude mice tumour formation MIA PaCa-2 cells were engineered to express inducible shRNA and *Sos WT , *Sos RA/LE or *Sos F929A constructs as described above. One million cells mixed equally with Matrigel (BD Biosciences) were injected (0.1 ml) subcutaneously into each flank of four 8-week-old female athymic nude mice NCr nu/nu (Taconic). After injection, mice were fed a diet containing doxycycline (1 g kg −1 ). When palpable, tumours were measured with a caliper every 3 days, and tumour volume was calculated by 0.5 × L × W 2 . When tumours reached a maximum volume (1500, mm 3 ), mice were euthanized and tumours were excised and photographed. To prepare lysates, tumour tissue was homogenized in RBD lysis buffer and then processed for immunoblot and GST-Raf-RBD pull-down assay. All mice were euthanized by 7 weeks post injection. All animal work was approved by New York University Langone Medical Centre Institutional Animal Care and Use Committee. Histology and immunohistochemistry Excised tumours were fixed with 10% buffered formalin, dehydrated in ethanol and then embedded with paraffin. For immunohistochemistry, 5μm-cut sections were deparaffinized, rehydrated in graded ethanol, quenched in 0.6% hydrogen peroxide/methanol for 15 min and antigens were boiled for 15 min in a microwave oven in 10 mM sodium citrate (pH 6.0) for antigen retrieval. Sections were blocked with 5% serum/1% bovine serum albumin/0.5% Tween-20 for 1 h. Slides were incubated with primary antibody (Ki-67 antibody, 0.8 μg ml −1 ) diluted in blocking buffer 1 h at room temperature. Following the primary antibody, slides were incubated with biotinylated secondary antibodies (Vector Laboratories) followed by ABC solution (Vector Laboratories) and developed with 3,3′-diaminobenzidine tetrahydrochloride for 15 min. Slides were counterstained with hematoxylin, dehydrated and mounted with Permount (Fisher). Slides were examined on a Nikon Eclipse 80i microscope. Statistical analysis Error bars of experiments performed in triplicate or more indicate s.d. Statistical calculations were performed with Microsoft Excel analysis tools. How to cite this article: Jeng, H-H. et al . Sos-mediated cross-activation of wild-type Ras by oncogenic Ras is essential for tumorigenesis. Nat. Commun. 3:1168 doi: 10.1038/ncomms2173 (2012).